Chloroplast-mediated activation of plant immune signalling inArabidopsis Chloroplasts have a critical role in plant immunity as a site for the production for salicylic acid and jasmonic acid, important mediators of plant immunity. However, the molecular link between chloroplasts and the cytoplasmic-nuclear immune system remains largely unknown. Here we show that pathogen-associated molecular pattern (PAMP) signals are quickly relayed to chloroplasts and evoke specific Ca 2+ signatures in the stroma. We further demonstrate that a chloroplast-localized protein, named calcium-sensing receptor (CAS), is involved in stromal Ca 2+ transients and responsible for both PAMP-induced basal resistance and R gene-mediated hypersensitive cell death. CAS acts upstream of salicylic acid accumulation. Transcriptome analysis demonstrates that CAS is involved in PAMP-induced expression of defence genes and suppression of chloroplast gene expression possibly through 1 O 2 -mediated retrograde signalling, allowing chloroplast-mediated transcriptional reprogramming during plant immune responses. The present study reveals a previously unknown chloroplast-mediated signalling pathway linking chloroplasts to cytoplasmic-nuclear immune responses. Plants are continuously exposed to a variety of biotic and abiotic stresses, and have evolved an intricate network of signal transduction pathways leading to transcriptome and metabolic reprogramming. Pathogen-associated molecular patterns (PAMPs) are recognized by pattern-recognition receptors in the plasma membrane and activate an array of basal defence responses (PAMP-triggered immunity, PTI), whereas pathogen-derived effector proteins trigger hypersensitive response (HR) cell death at the site of pathogen infection and confine the spread of pathogens (effector-triggered immunity, ETI) [1] . Plant immunity activates two parallel signal transduction pathways: cytoplasmic mitogen-activated protein kinase (MAPK) and Ca 2+ signalling pathways leading to transcriptional reprogramming, and a chloroplast-mediated pathway leading to the generation of chloroplast-derived reactive oxygen species (ROS) and the production of defence-related hormones, such as salicylic acid (SA) and jasmonic acid (JA) [2] . Possible involvement of chloroplasts in plant innate immunity has been discussed [3] . However, the molecular link between the chloroplast and cytoplasmic-nuclear immune signalling pathways remains largely unknown. In particular, it is not clear how immune signals are relayed to chloroplasts and how chloroplasts control the expression of nuclear-encoded defence genes. Extracellular stimuli evoke Ca 2+ signals in not only the cytoplasm, but also organelles such as mitochondria, peroxisomes and nuclei [4] , [5] . For example, the massive accumulation of Ca 2+ in mitochondria leads to the dysfunction of mitochondria and induction of apoptosis of mammalian cells [6] . However, very few studies have focused on Ca 2+ signals in chloroplasts. Calcium-sensing receptor (CAS) [7] is a thylakoid membrane-associated Ca 2+ -binding protein involved in the regulation of cytoplasmic Ca 2+ oscillations and extracellular Ca 2+ -induced stomatal closure [8] , [9] , [10] . Here we show that PAMP signals evoke a CAS-dependent transient Ca 2+ signal in chloroplasts, and that CAS is involved in transcriptional reprogramming through 1 O 2 -mediated retrograde signalling during plant innate immunity. This study is an important advancement in the understanding of cross talk between chloroplasts and the plant immune system. Biotic and abiotic stress-induced chloroplast Ca 2+ signals To measure the free Ca 2+ concentration in the stroma, the calcium-sensitive bioluminescent protein aequorin was targeted to the chloroplast stroma using an ribulose-1,5-bisphosphate carboxylase (RBCS) signal peptide ( Supplementary Fig. S1 ). As reported previously, stromal Ca 2+ was maintained at a very low concentration, as low as that in the cytoplasm ( Fig. 1a–f ), suggesting that Ca 2+ in chloroplasts is sequestered in the thylakoid lumen or by Ca 2+ -binding proteins [11] . We found that the bacterial PAMP flagellin peptide (flg22) induces a rapid Ca 2+ transient in the cytoplasm, followed by a long-lasting increase in the stromal free Ca 2+ level ( Fig. 1a ). A similar stromal Ca 2+ transient was also induced by the fungal PAMP chitin ( Fig. 1b ). On the other hand, control peptides induced no Ca 2+ signal in chloroplasts ( Supplementary Fig. S2a ). Furthermore, a flg22-induced stromal Ca 2+ transient was observed in transplastomic tobacco plants in which the aequorin gene had been integrated into the chloroplast genome ( Supplementary Fig. S2b ), confirming the occurrence of Ca 2+ dynamics in the chloroplast stroma. These findings demonstrate that extracellular PAMP signals are relayed rapidly to chloroplasts and evoke intrachloroplastic Ca 2+ transients. 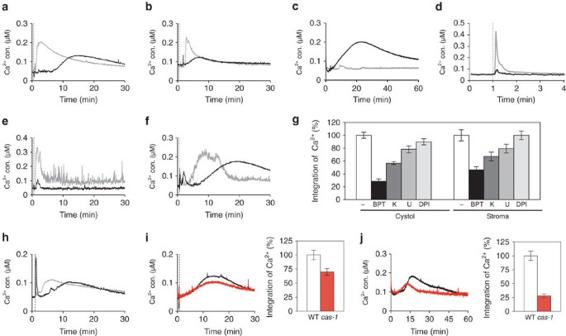Figure 1: Chloroplast Ca2+dynamics. (a–f,h) Aequorin (AEQ) luminescence from wild-type (WT) AEQ-expressing plants treated with (a) 1 μM flg22, (b) 100 μg ml−1chitin, (c) light-to-dark transition, (d) ice-cold MS medium, (e) 200 mM NaCl, (f) 500 mM sorbitol or (h) 30 μM ionomycin. The vertical dashed line indicates the time at which treatment was initiated. Experiments were repeated at least five times, with control treatments. Representative data are shown. Cytosolic and stromal Ca2+changes are indicated by grey and black lines, respectively. (g) Effects of signal transduction inhibitors on flg22-induced cytosolic and stromal Ca2+increase in WT AEQ-expressing plants. '−': no inhibitor, BPT: 5 mM 1,2-bis(2-aminophenoxy)ethaneN,N,N′,N′-tetraacetic acid (BAPTA), K: 2 μM K252a, U: 20 μM U-0126, DPI: 50 μM DPI. The time-integrated cytosolic or stromal Ca2+concentration upon 30-min treatment with 1 μM flg22 is shown. Data are the means±s.e.m. of relative values (n=4, control values were set of 100%). (i,j) Stromal Ca2+changes in WT (black lines, white bars) andcas-1knockout (red lines and bars) plants expressing AEQ. Plants were treated with (i) 1 μM flg22 or (j) light-to-dark transition. The integrated stromal Ca2+concentration was reduced incas-1compared with WT. Data are the means±s.e.m. of relative values (n=4). Figure 1: Chloroplast Ca 2+ dynamics. ( a – f , h ) Aequorin (AEQ) luminescence from wild-type (WT) AEQ-expressing plants treated with ( a ) 1 μM flg22, ( b ) 100 μg ml −1 chitin, ( c ) light-to-dark transition, ( d ) ice-cold MS medium, ( e ) 200 mM NaCl, ( f ) 500 mM sorbitol or ( h ) 30 μM ionomycin. The vertical dashed line indicates the time at which treatment was initiated. Experiments were repeated at least five times, with control treatments. Representative data are shown. Cytosolic and stromal Ca 2+ changes are indicated by grey and black lines, respectively. ( g ) Effects of signal transduction inhibitors on flg22-induced cytosolic and stromal Ca 2+ increase in WT AEQ-expressing plants. '−': no inhibitor, BPT: 5 mM 1,2-bis(2-aminophenoxy)ethane N , N , N ′, N ′-tetraacetic acid (BAPTA), K: 2 μM K252a, U: 20 μM U-0126, DPI: 50 μM DPI. The time-integrated cytosolic or stromal Ca 2+ concentration upon 30-min treatment with 1 μM flg22 is shown. Data are the means±s.e.m. of relative values ( n =4, control values were set of 100%). ( i , j ) Stromal Ca 2+ changes in WT (black lines, white bars) and cas-1 knockout (red lines and bars) plants expressing AEQ. Plants were treated with ( i ) 1 μM flg22 or ( j ) light-to-dark transition. The integrated stromal Ca 2+ concentration was reduced in cas-1 compared with WT. Data are the means±s.e.m. of relative values ( n =4). Full size image We further examined the effects of abiotic stresses on cytoplasmic and stromal Ca 2+ signals. Light-to-dark transition evoked a slow Ca 2+ transient in the stroma, but not the cytoplasm ( Fig. 1c ) [11] . We also found that other abiotic stresses induced stromal Ca 2+ transients in a stress-dependent manner. Cold and salt stresses elicited rapid stromal Ca 2+ spikes within a minute, whereas hyperosmotic stress induced a biphasic long-lasting Ca 2+ transient in the stroma ( Fig. 1d–f ). Stress-specific Ca 2+ signatures in the stroma may be involved in the regulation of photosynthesis and metabolic processes in response to the given stresses. In mammals, signal molecules such as staurosporine initially stimulate an increase in the cytoplasmic Ca 2+ concentration, and subsequently induce a mitochondrial Ca 2+ increase before apoptosis [6] . Similarly, PAMP-induced stromal Ca 2+ transients were always preceded by cytoplasmic Ca 2+ changes. We found that both chloroplastic and cytoplasmic Ca 2+ changes were markedly decreased by the extracellular Ca 2+ chelator 1,2-bis(2-aminophenoxy)ethane N , N , N ′, N ′-tetraacetic acid (BAPTA; Fig. 1g ). Furthermore, the Ca 2+ ionophore ionomycin induced a biphasic Ca 2+ increase in both the cytoplasm and the stroma ( Fig. 1h ). Interestingly, the second ionomycin-induced stromal Ca 2+ increase was preceded by the cytoplasmic Ca 2+ transient. From these results, we presume that PAMPs first induce Ca 2+ entry into the cytoplasm and, subsequently, the cytoplasmic Ca 2+ triggers a transient increase in the stromal Ca 2+ concentration. In addition, both the cytoplasmic and stromal Ca 2+ oscillations were partially reduced by inhibitors of serine/threonine protein kinase (K252a) and MAPKKs (U-0126), but not by an NADPH oxidase inhibitor (DPI; Fig. 1g ), suggesting the possible involvement of a MAP kinase cascade in the generation of cytoplasmic and stromal Ca 2+ signals. CAS is involved in chloroplast Ca 2+ signals CAS is a plant-specific thylakoid-associated Ca 2+ -binding protein [8] , [9] , [10] , [12] . To examine the possible role of CAS in the generation of stromal Ca 2+ transients, we measured flg22-induced stromal Ca 2+ transients in aequorin-expressing plants with a CAS knockout background ( cas-1 ). The aequorin-expressing cas-1 plants accumulated the same amount of aequorin protein as wild-type plants ( Supplementary Fig. S1a ). We found that flg22- and dark-induced long-lasting stromal Ca 2+ transients were markedly reduced in cas-1 ( Fig. 1i,j ), whereas cold-induced rapid stromal Ca 2+ spikes were not impaired in cas-1 ( Supplementary Fig. S3 ). Considering the localization of CAS in thylakoid membranes, CAS may be involved in Ca 2+ release from thylakoid membranes and the generation of a long-lasting stromal Ca 2+ signal. CAS is responsible for both PTI and ETI The presence of PAMP-induced Ca 2+ transients in the stroma underscores the importance of chloroplasts in plant immune signalling. We found that cas-1 plants exhibited severely impaired resistance to the virulent bacterium Pseudomonas syringae pv. tomato ( Pst ) strain DC3000 and to avirulent Pst DC3000 varieties ( Fig. 2a ). Surprisingly, PAMP (flg22)-induced defence-related events, such as stomatal closure ( Fig. 2b ), callose deposition ( Fig. 2c ) and accumulation of defence-related phenylpropanoids/flavonoids and their precursors ( Supplementary Fig. S4 ), were markedly compromised in cas-1 . Furthermore, flg22-induced PR1 and PR2 expression and stomatal closure were suppressed in two independent homozygous T-DNA insertion lines, cas-1 and cas-2 (ref. 8 ), whereas expression of CAS cDNA at wild-type levels in cas-1 restored flg22-induced PR1 and PR2 expression and stomatal closure ( Fig. 2d , Supplementary Fig. S5 ). These results demonstrate that the chloroplast protein CAS is involved in a range of basal defence responses. We further found that flg22-induced stomatal closure was impaired by the NADPH oxidase inhibitor diphenyleneiodonium (DPI) and by the nitric oxide (NO) scavenger 2-(4-carboxyphenyl)-4,4,5,5-tetramethylimidazoline-1-oxyl-3-oxide (cPTIO) in wild-type plants ( Fig. 2e ). On the other hand, exogenous application of hydrogen peroxide (H 2 O 2 ) or the NO donor sodium nitroprusside (SNP) could induce stomatal closure in cas-1 ( Fig. 2f ), suggesting that CAS acts upstream of ROS and NO signals in flg22-induced stomatal closure. 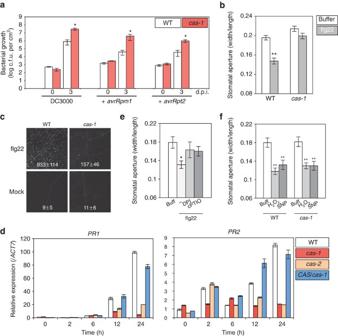Figure 2: Defects of immune regulation incas-1mutants. (a) Bacterial growth ofPseudomonas syringaepv.tomato(Pst) inArabidopsisleaves. Wild-type (WT) orcas-1plants were inoculated with virulent or avirulentPstDC3000 (OD600=0.0001), and numbers of bacteria per leaf area on days 0 and 3 were plotted on a log scale. Data are the means±s.e.m. of relative values (n=4; *P<0.05, Student'st-test). The experiment was repeated three times, with similar results; d.p.i., days post infection. (b) Flg22-induced stomatal closure. The stomatal aperture was calculated as the ratio of the pore width/guard cell length. Data are the means±s.e.m. of 50 stomata from three replicates (**P<0.01, Tukey-Kramer HSD test). (c) Detection of flg22-induced callose deposition with aniline blue. Representative pictures and the average number (with SD) of callose deposits per 4.5 mm2(n=8) are shown. The experiment was repeated three times, with similar results. (d) Flg22-induced gene expression was analysed by qRT–PCR at the indicated time points.ACT7was used as an internal standard. Data are means±s.e.m. of relative values (n=3). (e) Flg22-induced stomatal closure was inhibited in the presence of DPI or cPTIO. Leaves were pre-incubated with buffer (Buff) containing DPI or cPTIO for 30 min and then treated with 5 μM flg22 for 2 h. (f) Exogenously applied H2O2and SNP could induce stomatal closure incas-1. The stomatal aperture was calculated as the ratio of pore width/guard cell length. Data are the means±s.e.m. of 50 stomata (e: *P<0.05,f: **P<0.01, Tukey-Kramer HSD test). Figure 2: Defects of immune regulation in cas-1 mutants. ( a ) Bacterial growth of Pseudomonas syringae pv. tomato ( Pst ) in Arabidopsis leaves. Wild-type (WT) or cas-1 plants were inoculated with virulent or avirulent Pst DC3000 (OD 600 =0.0001), and numbers of bacteria per leaf area on days 0 and 3 were plotted on a log scale. Data are the means±s.e.m. of relative values ( n =4; * P <0.05, Student's t -test). The experiment was repeated three times, with similar results; d.p.i., days post infection. ( b ) Flg22-induced stomatal closure. The stomatal aperture was calculated as the ratio of the pore width/guard cell length. Data are the means±s.e.m. of 50 stomata from three replicates (** P <0.01, Tukey-Kramer HSD test). ( c ) Detection of flg22-induced callose deposition with aniline blue. Representative pictures and the average number (with SD) of callose deposits per 4.5 mm 2 ( n =8) are shown. The experiment was repeated three times, with similar results. ( d ) Flg22-induced gene expression was analysed by qRT–PCR at the indicated time points. ACT7 was used as an internal standard. Data are means±s.e.m. of relative values ( n =3). ( e ) Flg22-induced stomatal closure was inhibited in the presence of DPI or cPTIO. Leaves were pre-incubated with buffer (Buff) containing DPI or cPTIO for 30 min and then treated with 5 μM flg22 for 2 h. ( f ) Exogenously applied H 2 O 2 and SNP could induce stomatal closure in cas-1 . The stomatal aperture was calculated as the ratio of pore width/guard cell length. Data are the means±s.e.m. of 50 stomata ( e : * P <0.05, f : ** P <0.01, Tukey-Kramer HSD test). Full size image Some pathogens secret effector proteins ( Avr gene products) that suppress PTI. Conversely, effectors are recognized by plant proteins, which activate ETI leading to hypersensitive cell death at the infection site. We found that the cas-1 plants exhibited delayed and suppressed HR cell death compared with the wild type after inoculation with Pst DC3000 ( avrRpt2 ; Fig. 3a,b ). Interestingly, the Pst DC3000 ( avrRpt2 )-induced accumulation of ROS ( Supplementary Fig. S6a,b ) and NO ( Supplementary Fig. S6c,d ) was significantly reduced in cas-1 plants. Functional proof that CAS is a critical component in plant cell death was further demonstrated using virus-induced gene silencing (VIGS) in Nicotiana benthamiana plants. We cloned NbCAS from N. benthamiana ( Supplementary Fig. S7a ) and used VIGS to reduce its expression to <1% of the wild-type level ( Supplementary Fig. S7b ). NbCAS silencing resulted in a clear delay in the elicitor protein INF1-, the cf9/Avr9 elicitor/receptor- and the constitutively active N. tabacum MAP kinase kinase (NtMEK2 DD )-dependent cell death ( Fig. 3c,d , Supplementary Fig. S7c ), suggesting that CAS has a conserved role in plant cell death and may act downstream of the MAP kinase cascade in ETI. Considering a chloroplast localization of CAS, the above results suggest that chloroplasts might have critical roles in the positive regulation of plant immunity. 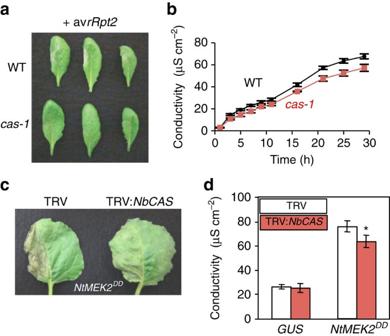Figure 3: CAS-dependent hypersensitive response (HR) cell death. (a,b) HR after inoculation with avirulentPseudomonas syringaepv.tomato(Pst) DC3000 (avrRpt2) (OD600=0.05). (a) HR lesions on the left side of leaves at 14 h. (b) Ion leakage after inoculation was measured at the indicated time points in leaves of wild-type (WT; black line) andcas-1knockout (red line) plants. Data are the means±s.e.m. of six discs from three replicates. (c)NbCAS-silencedN. benthamianaplants display a delay of cell death. Four- to five-week-oldNbCAS-silenced plants were infiltrated withAgrobacteriumcontaining theNtMEK2DDexpression vector. Tobacco rattle virus (TRV) was used as an experimental control. Pictures are taken at 3 days after inoculation. (d) Ion leakage at 3 days after infiltration withAgrobacteriumcontainingGUSorNtMEK2DDwas measured in silenced leaves. Data are the means±s.e.m. of six discs from three replicates. Significance was determined using Student'st-test (*P<0.05). Figure 3: CAS-dependent hypersensitive response (HR) cell death. ( a , b ) HR after inoculation with avirulent Pseudomonas syringae pv. tomato ( Pst ) DC3000 ( avrRpt2 ) (OD 600 =0.05). ( a ) HR lesions on the left side of leaves at 14 h. ( b ) Ion leakage after inoculation was measured at the indicated time points in leaves of wild-type (WT; black line) and cas-1 knockout (red line) plants. Data are the means±s.e.m. of six discs from three replicates. ( c ) NbCAS -silenced N. benthamiana plants display a delay of cell death. Four- to five-week-old NbCAS -silenced plants were infiltrated with Agrobacterium containing the NtMEK2 DD expression vector. Tobacco rattle virus (TRV) was used as an experimental control. Pictures are taken at 3 days after inoculation. ( d ) Ion leakage at 3 days after infiltration with Agrobacterium containing GUS or NtMEK2 DD was measured in silenced leaves. Data are the means±s.e.m. of six discs from three replicates. Significance was determined using Student's t -test (* P <0.05). Full size image CAS regulates SA biosynthesis It is unlikely that the compromised immunity of CAS knockout plants is caused by limited cellular resources, as cas-1 plants are photosynthetically competent [8] and do not show severe growth retardation ( Supplementary Fig. S8 ). Chloroplasts are involved in the biosynthesis of plant hormones such as SA, JA, abscisic acid (ABA), indole-3-acetic acid (IAA) and cytokinins (CKs). Thus, we examined the profiles of a set of plant hormones (SA, JA, ABA, IAA and CKs) during flg22-induced PTI. The accumulation of free SA was transiently induced by flg22 treatment within 6 h in wild-type plants, whereas JA and other hormones showed no significant change in levels ( Fig. 4a–e ), confirming a crucial role of SA in PTI signalling. Importantly, we found that CAS deficiency prevented flg22-induced accumulation of free SA ( Fig. 4a ) as well as glycosylated SA ( Supplementary Fig. S9 ). As the basal SA levels before flg22 treatment were normal in cas-1 plants, CAS is likely involved in the regulation of SA biosynthesis rather than the biosynthesis itself. SA is synthesized in chloroplasts via the chorismate pathway in Arabidopsis [13] . It has been shown that PAMPs induce SA biosynthesis in an ICS1-dependent manner [14] , [15] . Interestingly, the flg22-induced early expression of PAD4 , EDS5 , PBS3 and ICS1 , all of which are essential for SA biosynthesis, was significantly reduced in cas-1 plants before SA accumulation (~1 h; Fig. 4f ). On the other hand, PR1 expression was induced significantly by SA in cas-1 plants similarly to in wild-type plants ( Supplementary Fig. S10 ), indicating that the signal transduction pathways downstream of SA are independent of CAS. These results demonstrate that CAS is involved in flg22-induced SA biosynthesis through promoting the expression of nuclear-encoded SA biosynthesis genes. 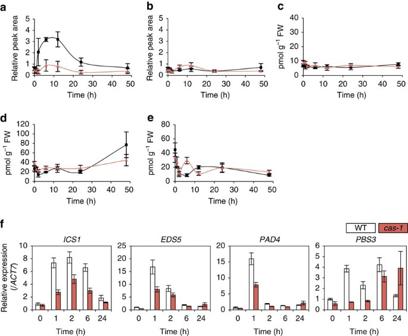Figure 4: CAS regulates salicylic acid (SA) biosynthesis and its related gene expression. (a–e) Flg22-induced phytohormone accumulation was measured at the indicated time points in leaves of wild-type (black line) andcas-1knockout (red line) plants. Data are the means±s.e.m. of three experiments. (a) SA and (b) jasmonic acid (JA) accumulation were measured using UPLC/TOFMS, and (c) abscisic acid (ABA), (d) indole-3-acetic acid (IAA) and (e) cytokinins were measured using nano-LC/MS/MS, and has been shown as the amount of hormones per fresh weight (FW) of plants. (f) Flg22-induced gene expression was analysed at indicated time points by qRT–PCR.ACT7was used as an internal standard. Data are mean±s.e.m. of three experiments. Figure 4: CAS regulates salicylic acid (SA) biosynthesis and its related gene expression. ( a – e ) Flg22-induced phytohormone accumulation was measured at the indicated time points in leaves of wild-type (black line) and cas-1 knockout (red line) plants. Data are the means±s.e.m. of three experiments. ( a ) SA and ( b ) jasmonic acid (JA) accumulation were measured using UPLC/TOFMS, and ( c ) abscisic acid (ABA), ( d ) indole-3-acetic acid (IAA) and ( e ) cytokinins were measured using nano-LC/MS/MS, and has been shown as the amount of hormones per fresh weight (FW) of plants. ( f ) Flg22-induced gene expression was analysed at indicated time points by qRT–PCR. ACT7 was used as an internal standard. Data are mean±s.e.m. of three experiments. Full size image CAS-dependent induction of nuclear-encoded defence genes These findings led us to hypothesize that CAS may be involved in chloroplast-to-nucleus retrograde signalling to control the expression of nuclear-encoded defence genes, including SA biosynthesis genes. Flg22 induces the expression of numerous defence-related genes in the nucleus [15] , [16] . To identify flg22-induced genes that are under the control of CAS, an Arabidopsis gene expression microarray (v4) was used to compare the flg22-induced transcription profiles of wild-type and cas-1 plants. We identified 687 upregulated and 1,235 downregulated genes in cas-1 plants treated with flg22 for 2 h ( Fig. 5a and Supplementary Data 1 and 2 ). By contrast, only 7 genes were upregulated and 197 genes were downregulated in non-treated cas-1 plants ( Fig. 5a and Supplementary Data 3 and 4 ). In all, 121 of the 197 downregulated and 6 of the 7 upregulated genes in non-treated cas-1 plants were also down- and upregulated in flg22-treated cas-1 plants, respectively. Quantitative reverse transcription–PCR (qRT–PCR) confirmed the array results for selected targets ( Figs 4f and 5c ). Interestingly, the expressions of one-third (827 genes) of the flg22-induced early genes (within 3 h) [17] were suppressed in cas-1 ( Fig. 5a,b , Supplementary Fig. S11 ). Similarly, two-thirds of genes downregulated in flg22-treated cas-1 were flg22-induced in wild type. Furthermore, the 403 genes upregulated in flg22-treated cas-1 were enriched for genes that were suppressed by flg22 in wild type (58.7%). Gene expression analysis using the Expression Browser at Bio-Array Resource (BAR) [18] showed that genes downregulated in flg22-treated cas-1 were also enriched in NPP1- and HrpZ-responsive genes, as well flg22-responsive genes ( Supplementary Fig. S12a ). CAS, therefore, likely has a universal role in PAMP-induced gene expression. 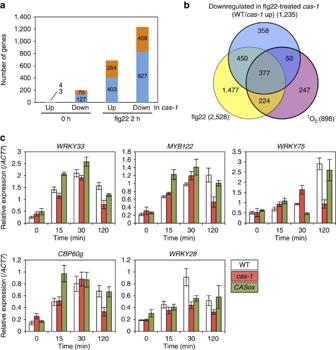Figure 5: Genome-wide transcriptional analysis ofcas-1mutants in flg22-induced immunity. (a) Numbers of differentially expressed genes that were up- or downregulated incas-1plants treated with flg22 for 2 h (right) or not treated (left). Genes that were regulated by flg22 within 3 h are shown in blue. Several flg22-induced genes were downregulated before flg22 treatment incas-1plants. (b) Venn diagram showing the overlap of downregulated genes in flg22-treatedcas-1(WT/cas-1up: blue), flg22-induced genes within 3 h (flg22: yellow) and chloroplastic1O2-dependent genes under light for 2 h in theflumutant background (1O2: purple). (c) Expression of flg22-induced genes was analysed at indicated time points by qRT–PCR to confirm microarray experiments.ACT7was used as an internal standard. Data are mean±s.e.m. of three experiments. WT, wild type. Figure 5: Genome-wide transcriptional analysis of cas-1 mutants in flg22-induced immunity. ( a ) Numbers of differentially expressed genes that were up- or downregulated in cas-1 plants treated with flg22 for 2 h (right) or not treated (left). Genes that were regulated by flg22 within 3 h are shown in blue. Several flg22-induced genes were downregulated before flg22 treatment in cas-1 plants. ( b ) Venn diagram showing the overlap of downregulated genes in flg22-treated cas-1 (WT/ cas-1 up: blue), flg22-induced genes within 3 h (flg22: yellow) and chloroplastic 1 O 2 -dependent genes under light for 2 h in the flu mutant background ( 1 O 2 : purple). ( c ) Expression of flg22-induced genes was analysed at indicated time points by qRT–PCR to confirm microarray experiments. ACT7 was used as an internal standard. Data are mean±s.e.m. of three experiments. WT, wild type. Full size image Gene ontology analysis using the Arabidopsis Classification Super Viewer demonstrated a significant over-representation of 'response to stress' (3.04-fold, P =5.33E−50), 'response to abiotic and biotic stimulus' (2.49-fold, P =2.83e–28) and signal transduction (2.26-fold, P =7.17e–14) categories among the flg22-treated cas-1 downregulated genes ( Supplementary Fig. S12b–e ). The downregulated genes included a number of GTPase, Ca 2+ signalling and SA signalling genes ( Supplementary Data 5 ). CAS was also required for flg22-induced expression of CYP79B2 , CYP79B3 and PAD3 genes for cytochrome P450 that are essential for the production of camalexin, the charateristic phytoalexin of Arabidopsis . On the other hand, the flg22-treated cas-1 upregulated genes were enriched for those involved in 'electron transport or energy pathways' (2.34-fold, P =1.34e–3). Interestingly, genes for plastid (1.93-fold, P =1.46e–5) and chloroplast (1.86-fold, P =5.29e–12) proteins were significantly enriched among the upregulated genes in flg22-treated cas-1 . These results suggest that chloroplasts may promote defence gene expression and suppressing chloroplast (photosynthesis) gene expression through CAS during PTI. Chloroplast regulation of nuclear transcriptional programmes We identified 99 and 78 transcription factor (TF) genes among the downregulated and upregulated genes in cas-1 , respectively. WRKYs are a large family of plant-specific TFs (with 72 genes in Arabidopsis ) that act mainly in the defence response network of plant cells [19] , [20] . We identified one-third of WRKY genes under the control of CAS (25 downregulated and 1 upregulated; Supplementary Data 1 ), suggesting an important role for WRKYs in CAS-dependent PTI. In fact, the most represented motif in the promoters (500-bp upstream regions) of the flg22-treated cas-1 downregulated genes was TTGAC ( Supplementary Table S1 ). TTGAC is part of the W-box consensus sequence (TTGAC[C/T]) of the WRKY-binding site [19] . The W-box motif was found in the promoters of 539 of the 1,235 genes downregulated in flg22-treated cas-1 (44%). The W-box sequences were enriched in the promoter region at 200–400 bp upstream of the translation start site ( Supplementary Fig. S13 ), confirming the W-box as a cis -element of the flg22-treated cas-1 downregulated (CAS-dependent) genes. The flg22-treated cas-1 downregulated TFs included several key factors, such as WRKY33 relaying the MAPK signal to the transcription network in PTI [19] , and WRKY28 / WRKY46 (ref. 21 ) and CBP60g / SARD1 (ref. 22 ), essential for the activation of ICS1 and SA synthesis. Taken together, WRKY TFs might have a critical role in PAMP (flg22)-induced chloroplast-mediated transcriptional reprogramming in plant innate immunity. By contrast, the upregulated TF genes included AtGLK2 (ref. 23 ), CIA2 (ref. 24 ), GATA21 ( GNC ) [25] and a set of chloroplast sigma factors ( AtSIG1 , AtSIG3 , AtSIG4 and AtSIG6 ), which are required for chloroplast development [26] . Interestingly, the I-box motif involved in light-responsive photosynthetic gene expression [27] was found in the promoters of 149 of the 687 genes upregulated in flg22-treated cas-1 plants. Thus, it seems that chloroplasts (CAS) regulate plant immune responses through activation of defence-related TFs and suppression of chloroplast function/development by inactivating TFs required for chloroplast development. Chloroplast-derived ROS and CAS-dependent gene expression To examine the role of flg22-induced TFs during early PTI, we performed a time course expression analysis using qRT–PCR. PAMP (flg22) triggered a rapid (within 15 min) and transient increase in the expression of TF genes such as CBP60g , WRKY28 , WRKY33 and MYB122 ( Fig. 5c ), suggesting a role for them in early transcriptional reprogramming during PTI. On the other hand, the expression of WRKY75 ( Fig. 5c ) and SA biosynthesis-related genes ( Fig. 4f ) peaked at 1–2 h, and PR1 gene expression was induced after 12 h. Interestingly, flg22-induced early expression of TF genes (within 30 min) was not suppressed in cas-1 mutants, but CAS was needed for the middle phase (1–2 h) expression of TF ( Fig. 5c ) and SA biosynthesis-related genes ( Fig. 4f ), and PR1 gene expression at the late phase (24 h). On the other hand, overexpression of CAS hastened and enhanced early expression of a set of TF genes such as CBP60g , WRKY33 and MYB122 ( Fig. 5c ), suggesting a possible activating role of CAS in defence-related TF gene expression. These results imply that after a ~30-min lag chloroplasts may generate CAS-dependent retrograde signals, which is required for prolonged expression of the early defence-related TFs and promotes subsequent expression of defence-related genes. It has been proposed that chloroplast-derived ROS signals, such as 1 O 2 and H 2 O 2 , may activate the expression of nuclear-encoded defence genes [28] , [29] . Notably, we found that 427 of 1,235 genes downregulated in flg22-treated cas-1 overlapped with genes that were 1 O 2 -responsive in the flu mutant (fold change >3.0), including several 1 O 2 marker genes, EDS5 and ERD1 ( Fig. 5b and Supplementary Data 1 ) [29] . By contrast, only 153 genes overlapped with methyl viologen (MV)-induced O 2 − /H 2 O 2 -responsive genes (fold change >3.0; Supplementary Data 1 ) [30] . These results suggest a role for CAS in 1 O 2 signalling to control nuclear-encoded defence gene expression. CAS is a plant-specific low-affinity/high-capacity non-EF-hand Ca 2+ -binding protein that is associated with thylakoid membranes of chloroplasts ( Supplementary Fig. S14 ) [8] , [9] , [10] , [12] . This study demonstrates that the chloroplast protein CAS is required for both PTI and R gene-mediated ETI. PTI and ETI are controlled by complex interconnected signalling networks including the MAP kinase cascade, ROS signalling and the plant hormones SA, JA and ethylene [1] , [2] . We found that CAS may act upstream of ROS signalling in PAMP-induced stomatal closure, and downstream of the MAP kinase cascade and upstream of ROS/NO in ETI ( Figs 2f , 3c and Supplementary Fig. S6 ). Furthermore, we demonstrated that CAS is required for the flg22-induced accumulation of SA ( Fig. 4 ). Considering the chloroplast localization of CAS, these findings suggest that chloroplasts have a critical role in both PTI and ETI. CAS may be involved in the coupling of chloroplasts and cellular immune responses and may function upstream of ROS signalling and SA biosynthesis. We found that CAS is required for transcriptional activation of SA biosynthesis genes, such as ICS1 , EDS5 , PBS3 and PAD4 , whereas the SA signalling pathway downstream of SA is not impaired in cas-1 plants ( Fig. 4 and Supplementary Fig. S10 ). Furthermore, microarray analysis revealed that the expression of a set of TF genes ( WRKY28 / WRKY46 and CBP60g / SARD1 ) [21] , [22] , essential for activation of SA biosynthesis genes, was greatly reduced in cas-1 plants ( Supplementary Data 1 ). These results suggest that CAS mediates the chloroplast control of SA biosynthesis through these TFs, and the resultant SA subsequently induces a range of basal defence responses. On the other hand, considering the co-localization of CAS and SA biosynthesis in chloroplasts, there remains a possibility that CAS might directly modulate ICS1 activity within chloroplasts. Recognition of pathogens results in a massive reprogramming of plant cells to activate defence responses and reduce other cellular activities, such as cellular development/organization and photosynthesis [31] . Microarray analysis demonstrates that CAS controls transcriptional reprogramming during PTI through activation of defence-related TFs including a number of WRKYs and suppression of TFs involved in chloroplast development. We found that a short DNA motif, W-box (TTGAC[T/C]), is over-represented in the promoter sequences of flg22-treated cas-1 downregulated (CAS-dependent flg22-induced) genes (52.6%). The WRKY family TFs regulate biotic and abiotic stress responses and share the WRKY domain that recognizes the W-box [19] . Interestingly, the W-box is over-represented not only in the promoter regions of defence-related genes, but also in O 3 -responsive [32] and superoxide-responsive promoters [30] . On the other hand, some promoters of CAS-dependent flg22-suppressed genes contain an I-box motif, a common cis -element characteristic of photosynthesis genes ( Supplementary Table S1 ) [27] . Thus, these results suggest that CAS-dependent defence gene expression might be mediated by WRKY TFs that target W-box-containing promoters of plant defence genes in a ROS-dependent manner, whereas CAS may control PAMP-induced suppression of photosynthesis gene expression via an I-box-binding protein/I-box-mediated transcription system. Interestingly, some TF genes occur more rapidly in CAS-overexpressing plants, suggesting a direct role for CAS in the promotion of defence-related TF gene expression. However, the molecular function of CAS remains largely unknown. CAS deficiency may disrupt unidentified chloroplast function related to defence responses and indirectly affect the expression pattern of flg22-induced defence genes. Nevertheless, these findings strongly suggest that chloroplasts have a critical role in the transcriptional regulation of plant immune signalling. It has been proposed that chloroplast-derived retrograde signals, such as chlorophyll synthesis intermediates and chloroplast-derived ROS, control the expression of nuclear-encoded genes for photosynthesis and defence responses [33] , respectively. When the cell is unable to dissipate excess excitation energy, chloroplasts generate ROS, such as singlet oxygen ( 1 O 2 ) or hydrogen peroxide (H 2 O 2 ), which activate distinct sets of genes. Interestingly, 1 O 2 triggers a cell death programme that resembles the effector-triggered HR [34] . Here, we found that almost one-third of CAS-dependent flg22-induced genes are also induced by 1 O 2 in the flu mutant ( Fig. 5b ), but not by MV-induced H 2 O 2 . Furthermore, CAS-dependent flg22-induced genes also overlap with the light-induced genes in flu mutants overexpressing thylakoid-localized ascorbate peroxidase, which is expected to compensate for chloroplast-derived O 2 − and H 2 O 2 , but not 1 O 2 (ref. 29 ). These results suggest a role for chloroplast-derived 1 O 2 signalling in CAS-dependent transcriptional control of nuclear-encoded defence genes. Moreover, the flg22-induced extracellular ROS burst was not impaired in cas-1 plants ( Supplementary Fig. S15 ), suggesting a limited role of NADPH oxidase-derived O 2 − and H 2 O 2 in CAS-dependent immune responses. In addition, it has been recently shown by another group that extracellular Ca 2+ -induced generation of chloroplast NO and ROS is dependent on CAS, but not plasma membrane-localized NADPH oxidase [35] , providing further confirmation of the role of CAS in ROS production in chloroplasts. Thus, we assume that CAS may be involved in the chloroplast-derived 1 O 2 -mediated retrograde signalling that regulates the expression of nuclear-encoded defence-related genes at an early stage in PTI. In fact, the release of 1 O 2 in the flu mutant triggers the expression of WRKY33 and WRKY46 TFs during the first 30 min of reillumination [36] , a subsequent drastic increase in free SA levels, and the expression of PR1 and PR5 genes [37] . Time course qRT–PCR analysis revealed that chloroplasts generate signal(s) after a 30-min lag time. Interestingly, it has been reported that Cle elicitor induces 1 O 2 in cultured cells after a 10-min lag period, and peaks at 30 min after the treatment [38] . This time course coincides well with those of flg22-induced defence-related gene expression and subsequent SA biosynthesis. We propose that a CAS-dependent chloroplast-derived signal (possibly 1 O 2 ) may modulate the defence responses through transcriptional reprogramming of defence-related genes. Therefore, it is speculated that pathogen signals are transmitted to chloroplasts before the production of chloroplast-derived ROS signal(s). Sai and Johnson [11] previously reported that light-to-dark transition triggers a transient rise of stromal free Ca 2+ levels in tobacco chloroplasts. Here, we show that PAMPs evoke a long-lasting stromal Ca 2+ increase following a rapid cytoplasmic Ca 2+ transient ( Fig. 1a,b ). It is known that the thylakoid lumen accumulates Ca 2+ at a high level. CAS is responsible for the full activation of long-lasting stromal Ca 2+ transients induced by flg22 and darkness ( Fig. 1i,j ). Thus, it is plausible that CAS regulates the release and/or uptake of Ca 2+ through thylakoid membranes to evoke long-lasting stromal Ca 2+ signals. We further demonstrate that several abiotic stresses also induce stress-specific stromal Ca 2+ signals ( Fig. 1d–f ), suggesting that stromal Ca 2+ signatures may be involved in stress-specific responses, including rapid inhibition of photosynthesis and accumulation of JA [39] , [40] . Interestingly, chloroplasts contain several EF-hand Ca 2+ sensor proteins and other types of Ca 2+ -binding proteins [41] . PAMP-induced stromal Ca 2+ transients precede CAS-dependent defence gene expression and SA biosynthesis, suggesting a role for chloroplast Ca 2+ signatures in the activation of defence gene expression. Interestingly, genes induced by some abiotic stimuli such as light-to-dark transition and osmotic stress, which evoke long-lasting stromal Ca 2+ signals, were enriched among genes downregulated in flg22-treated cas-1 , but cold and salt-induced genes were not ( Supplementary Fig. S16 ). The W-box sequences were also over-represented in the promoter regions of genes upregulated by osmotic stress, but not of cold and salt stimili-induced genes ( Supplementary Tables S1 and S2 ). Thus, chloroplast Ca 2+ signatures are likely involved in stress-specific gene expression. It has been shown that Ca 2+ regulates FBPase [42] , [43] , and the stability of the photosystem II and thylakoid O 2 evolving complexes [44] . The stromal Ca 2+ transients coincide with the stress-induced rapid downregulation of photosynthesis [39] , [45] , [46] . Importantly, photosynthesis collapse may lead to photo-induced production of ROS including 1 O 2 (ref. 47 ). Taken together, long-lasting stromal Ca 2+ signals may induce the downregulation of photosynthetic electron flow, leading to the production of ROS. Interestingly, cas-1 mutants show higher values of non-photochemical chlorophyll fluorescence quenching than do wild-type plants [8] . Non-photochemical chlorophyll fluorescence quenching has a major role in the protection of the photosynthetic apparatus against damage by excess light and the production of ROS [48] . Herein, we demonstrated a novel chloroplast-dependent pathway that controls plant innate immunity through stromal Ca 2+ signalling and chloroplast-to-nuclei retrograde ROS signalling ( Fig. 6 ). Recent studies have shown that plant innate immune responses are modified by light and intrinsic circadian cues [49] , [50] . Chloroplasts may act as an environmental sensor in plants [51] . Interestingly, CAS is required for photoacclimation in Chlamydomonas [12] . Furthermore, CAS has been shown to be involved in the coupling of diurnal extracellular Ca 2+ oscillations to cytosolic Ca 2+ oscillations [52] . Characterization of the molecular function of CAS and chloroplast Ca 2+ signalling would provide insight into the role of chloroplasts in cross talk among environmental regulation pathways and plant immunity. 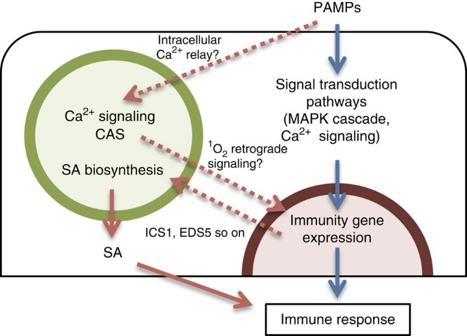Figure 6: Molecular cross talk between chloroplasts and cytoplasmic-nuclear immune system. Pathogen-associated molecular pattern (PAMP) signals are quickly relayed to chloroplasts and evoke specific Ca2+signatures in the stroma. The thylakoid-associated calcium sensor protein CAS is involved in the generation of chloroplast Ca2+signals. CAS is also essential for the induction of PAMP-induced defence genes, including salicylic acid (SA) biosynthesis genes, possibly through singlet oxygen (1O2)-mediated retrograde signalling, Thus, SA-mediated immune responses are dependent on CAS. Chloroplast-mediated pathways involved in the communication between chloroplasts and the cytoplasmic-nuclear signal transduction pathways are shown as dotted red arrows. The cytoplasmic and SA-mediated immune pathways are shown as red and blue arrows, respectively. Figure 6: Molecular cross talk between chloroplasts and cytoplasmic-nuclear immune system. Pathogen-associated molecular pattern (PAMP) signals are quickly relayed to chloroplasts and evoke specific Ca 2+ signatures in the stroma. The thylakoid-associated calcium sensor protein CAS is involved in the generation of chloroplast Ca 2+ signals. CAS is also essential for the induction of PAMP-induced defence genes, including salicylic acid (SA) biosynthesis genes, possibly through singlet oxygen ( 1 O 2 )-mediated retrograde signalling, Thus, SA-mediated immune responses are dependent on CAS. Chloroplast-mediated pathways involved in the communication between chloroplasts and the cytoplasmic-nuclear signal transduction pathways are shown as dotted red arrows. The cytoplasmic and SA-mediated immune pathways are shown as red and blue arrows, respectively. Full size image Plant materials and growth conditions Arabidopsis thaliana wild-type Columbia ecotype, CAS knockout mutants ( cas-1 and cas-2 ) [8] , CAS-overexpressing plants [8] and apoaequorin transgenic plants were germinated and grown on one-half Murashige and Skoog (MS) medium containing 0.8% (w/v) agar at 22 °C with 16-h light (80–100 μmol m −2 s −1 )/8-h dark cycles for 2–4 weeks. For pathogen inoculation experiments, 4- to 5-week-old wild-type and cas-1 plants grown on soil with 10-h light (140–160 μmol m −2 s −1 )/14-h dark cycles were used. Measurements of cytosolic and stromal Ca 2+ concentrations Ca 2+ measurements were performed as previously described, with some modifications [8] . Detached rosette leaves from plate-grown transgenic wild-type and cas-1 Arabidopsis plants expressing aequorin were floated on one-half MS liquid medium containing 5 μM coelenterazine, then kept overnight at 22 °C in the dark. Aequorin luminescence was measured with Lumi Counter 2500 (Microtec). The amount of reconstituted aequorin in the plants was determined by the addition of an equal volume of 2 M CaCl 2 in 20% ethanol at the end of the measurements. Aequorin luminescence calibration was performed as previously described [53] . Elicitor peptide flg22 was synthesized by Biologica(Nagoya). The chitin suspension was prepared as previously described [54] . Chitin (Wako) was hydrolysed with concentrated HCl, and left for 2 h at room temperature with occasional mixing. The hydrolysed chitin was then washed with water twice, and dissolved in one-half MS medium to achieve a final chitin concentration of 1.0 mg ml −1 . Cold shock stress was applied to the plants by adding ice-cold one-half MS medium to a leaf floated in a cuvette. The measurement of dark-stimulated Ca 2+ changes was performed as described [11] . Ten-day-old plants were incubated at 22 °C under 24-h light conditions (22 μmol m −2 s −1 ), and then transferred to the dark. In pharmacological experiments, BAPTA (Wako), K-252a (Wako), U-0126 (Calbiochem) or DPI (Calbiochem) were dissolved in ethanol or DMSO and applied to plants in a cuvette at the appropriate concentration and left for 30 min before treatment with flg22. Plant inoculation and quantification of bacteria Pathogen inoculations, bacterial growth counts and ion conductance measurements were performed as previously described, with some modifications [55] . The virulent strain of Pst DC3000 and avirulent strains of Pst DC3000 (carrying avrRpt2 or avrRpm1 ) were cultured at 28 °C in King's B medium containing 25 μg ml −1 kanamycin, 100 μg ml −1 rifampicin and 50 μg ml −1 cycloheximide, washed once in 10 mM MgCl 2 and resuspended in 10 mM MgCl 2 . Needleless syringe infiltration was used to inoculate plants with pathogen in all cases. Immediately after the infiltration, the plants were allowed to dry and were then kept under 100% humidity for the remainder of the experiment. At indicated time points, leaf discs were collected, ground to homogeneity in water and the titre was determined by serial dilution and plating. For measurements of ion leakage, 6 leaf discs (8-mm diameter) were removed immediately following infiltration ( t =0) and floated in 25 ml of water. After 30 min, the water was removed and replaced with 10 ml of new water. The conductance of this water was measured at the indicated time points. Stomatal aperture measurements Stomatal aperture measurements were performed as previously described [8] . Rosette leaves from 3- to 4-week-old plate-grown plants were detached and floated on the incubation buffer (10 mM 2-(N-morpholino)ethanesulfonic acid (MES)–KOH, pH 6.15; 10 mM KCl; 50 μM CaCl 2 ) for 2 h at 22 °C, in 80–100 μmol m −2 s −1 light. After 2 h, the leaves in the incubation buffer were treated with or without 5 μM flg22, 10 μM H 2 O 2 or 50 μM SNP and then incubated for an additional 2 h. For inhibitor experiments, the leaves were pre-incubated with 50 μM DPI or 200 μM cPTIO for 30 min before treatment with flg22. After the incubation period, epidermal strips of the leaves were observed by microscopy. The stomatal aperture was calculated as the ratio of the pore width/guard cell length. A guard cell length of 22–28 μm was used in the experiments. Callose deposition Rosette leaves of 4- to 5-week-old soil grown wild-type and cas-1 plants were infiltrated with 10 mM Tris–HCl (pH 7.2; mock) or the same solution containing 5 μM flg22. After 24 h, the leaves were detached, cleared with ethanol and stained with 10 mM Tris–HCl (pH 7.2) containing 0.01% aniline blue for 30 min. Leaves were stored in 50% glycerol and observed via epifluorescence microscopy under UV illumination with a broadband DAPI filter set. Measurements of callose deposition were made using the image-processing software IMAGEJ. Metabolite analysis by nano-LC/MS/MS and UPLC/TOFMS Levels of SA, JA, ABA, IAA, zeatin and zeatin riboside were analysed by nano-liquid chromatography ?" tandem mass spectrometry (LC/MS/MS) with a modification of the methods described by Izumi et al . [56] . Briefly, 100 mg of leaf samples were homogenized using a ballmill and extracted with methanol/H 2 O/formic acid (75:20:5) solution containing internal standards (40 pmol (d 7 -DHZOG, d 3 -DHZR, d 6 -iP, d 6 -iPR), 200 pmol (d 6 -ABA), 400 pmol (d 3 -DHZ), 1,000 pmol (d 2 -GA 1 , d 5 -IAA, d 2 -GA 7 ), 2 μmol lidocaine and 10 μmol (+)-10-camphorsulfonic acid). After centrifugation, half of the supernatant was used for analyses of SA, JA and small charged molecules by ultra-performance liquid chromatography - time-of-flight mass spectrometry (UPLC/TOFMS) as described previously [56] , [57] . The remaining supernatant was extracted with water and dried. The dried samples were dissolved in 1 M formic acid and applied to the OASIS MCX cartridge. The fraction containing ABA and IAA was eluted with methanol and, subsequently, the CK fraction was eluted with 60% methanol solution containing 0.35 M NH 4 . Eluted fractions were further purified and analysed by nano-LC/MSMS. SA was also measured using a conventional high-performance liquid chromatography system. A total of 200 mg of seedling samples without roots was homogenized and extracted with 100% methanol containing the internal standard anisic acid. Free and glycosylated SA were separated and analysed by high-performance liquid chromatography. VIGS and Agrobacterium -mediated transient expression VIGS was done as described by Ratcliff et al . [58] . pBINTRA6 (RNA1) and the pTV00 containing the NbCAS cDNA fragment (RNA2) were transformed by electroporation separately into Agrobacterium tumefaciens strain GV3101 (pSoup). A mixture of equal parts of Agrobacterium suspensions of RNA1 and RNA2 was infiltrated into 2- to 3-week-old N . benthamiana leaves. For cell death assay, Agrobacterium strain GV3101 (pSoup) carrying NtMEK2 DD , INF1 , cf9 / Avr9 or GUS (pGreen binary vectors) was infiltrated into the upper leaves of 4- to 5-week-old NbCAS -silenced N. benthamiana plants. Microarray experiments and data analysis The genome-wide microarray analyses were performed using the Arabidopsis v4 2 colour microarray (Agilent Technologies). Light grown, 2-week-old, wild-type and cas-1 mutant plants were floated on one-half MS medium for 1 day (0 h), and then treated with 1 μM flg22 for 2 h. Total RNA was isolated with the Qiagen RNeasy plant mini kit following the manufacturer's instructions. Two independent biological replicates were performed for each sample and control. Each 200-ng total RNA sample was used to prepare Cy3- or Cy5-labelled target cRNA with the Low Input Quick Amp Labeling Kit (Agilent Technologies) and used in dual colour microarray hybridization with the Agilent Arabidopsis v4 oligo microarray slide. A dye-swap experiment was performed with two different RNA populations to eliminate the signal variation caused by the differential labelling efficiency of Cy3 and Cy5 dyes. The microarray data were normalized by the LOWESS method using the Feature Extraction software v. 10.7 (Agilent Technologies) and the expression ratios were analysed (Non-Uniformity Outlier and Feature Population Outlier). Data with a P -value of >0.01 were eliminated. The genes that showed a consistent expression pattern in cas-1 and at least a twofold difference in the expression level in both slides are listed in Supplementary Data 1 . The genes induced by flg22 (ref. 17 ), by illumination of the flu mutant (chloroplast-derived 1 O 2 ) [29] and the flu mutant overexpressing thylakoid-localized ascorbate peroxidase [29] and by MV [30] were obtained from publications. To extract flu -regulated genes, raw signal intensity data (GSE10812) were obtained from the NCBI GEO database [29] . The genes that revealed a consistent expression pattern at 2 h after a dark-to-light shift in the flu mutant compared with wild type and exhibited at least a threefold difference in the expression level were used for this analysis. Gene ontology and promoter sequence analyses Gene ontology analysis was performed with the Arabidopsis Classification SuperViewer at the BAR of the University of Toronto. We compared the gene expression profiles of our microarray experiments with available expression data via the expression browser at BAR. We also searched for over-represented cis -elements in the 500-bp upstream regions of the down- and upregulated genes in flg22-treated cas-1 plants using the Regulatory Sequence Analysis tool (RSAT; http://rsat.ulb.ac.be/rsat ). Accession codes: The NbCAS sequence has been deposited in the DNA Data Bank of Japan under accession code AB720027 . How to cite this article: Nomura, H. et al . Chloroplast-mediated activation of plant immunity signalling in Arabidopsis . Nat. Commun. 3:926 doi: 10.1038/ncomms1926 (2012).